Direct induction of haematoendothelial programs in human pluripotent stem cells by transcriptional regulators Advancing pluripotent stem cell technologies for modelling haematopoietic stem cell development and blood therapies requires identifying key regulators of haematopoietic commitment from human pluripotent stem cells (hPSCs). Here, by screening the effect of 27 candidate factors, we reveal two groups of transcriptional regulators capable of inducing distinct haematopoietic programs from hPSCs: pan-myeloid (ETV2 and GATA2) and erythro-megakaryocytic (GATA2 and TAL1). In both cases, these transcription factors directly convert hPSCs to endothelium, which subsequently transform into blood cells with pan-myeloid or erythro-megakaryocytic potential. These data demonstrate that two distinct genetic programs regulate the haematopoietic development from hPSCs and that both of these programs specify hPSCs directly to haemogenic endothelial cells. In addition, this study provides a novel method for the efficient induction of blood and endothelial cells from hPSCs via the overexpression of modified mRNA for the selected transcription factors. Human pluripotent stem cells (hPSCs), both embryonic stem cells (hESCs) and induced PSCs (hiPSCs), offer a plentiful source of blood cells for experimentation and therapeutic purposes. Although significant advances have been made in haematopoietic differentiation from hPSCs, a better understanding of the key regulators of haematopoietic commitment is required to achieve the scalability of production of blood cells from hPSCs and to enable de novo generation of haematopoietic stem cells (HSCs). Transcription factors (TFs) have been recognized as critical regulators of early embryonic development. TFs function as key elements of a gene regulatory network that guide the acquisition of specific properties by particular cell type [1] . Several TFs are identified as master regulators of haematopoietic development in the mouse embryo [2] , [3] , [4] , [5] . Many of them are also involved in the regulation of endothelial development, reflecting a close developmental link between endothelial and haematopoietic cells [6] . In fact, recent studies have demonstrated that in the embryo, haematopoietic cells including HSCs arise from endothelial cells with blood-forming potential, haemogenic endothelium [7] , [8] , [9] , indicating that blood development proceeds through an endothelial intermediate stage. To unravel the most essential TFs required for the induction of the blood programme from hPSCs, we performed comprehensive gain-of-function screening. Using this approach, we identified two optimal combinations of TFs capable of inducing distinct, robust haematopoietic programs from PSCs: pan-myeloid (ETV2 and GATA2) and erythro-megakaryocytic (GATA2 and TAL1). Interestingly, both TF combinations directly induced haemogenic endothelial cells, which subsequently transformed into blood progenitors with a distinct spectrum of haematopoietic differentiation. These results suggest, firstly the specification to discrete types of haematopoietic progenitors begins at the haemogenic endothelium stage and is regulated by distinct transcriptional programs, and secondly, only a few TFs are sufficient to activate the haematoendothelial programme from hPSCs, and trigger in a culture dish the sequence of events observed during blood development in the embryo. Also presented, is a novel approach to induce the efficient production of endothelium and blood from hPSCs using mmRNA. Selection of candidate genes and screening system design To induce the haematopoietic programme in hPSCs, we first assembled a list of candidate transcriptional regulators involved in mesodermal and angiohaematopoietic specification and HSC development through literature review. To prioritize genes for screening, we used molecular profiling data obtained from the analysis of the gene expression of hESC-derived mesodermal and vascular progenitors with or without haematopoietic potential we identified in our prior studies [10] , [11] . On the basis of these data, we selected 27 genes ( Supplementary Fig. 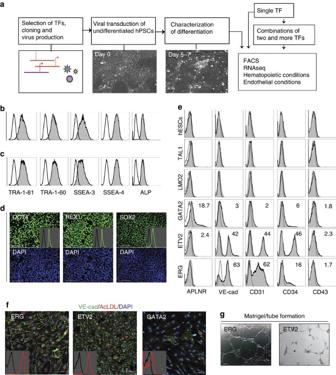Figure 1: Gain-of-function screening in hPSCs. (a) Schematic diagram of the screening system; (b–d) Flow cytometric and immunofluorescent analysis of expression of pluripotency markers in H1 hESCs growing on matrigel for 5 days in standard conditions in mTeSR1 medium (b) and basal growth-factor free TeSR1 medium containing 100 ng ml−1SCF, 50 ng ml−1TPO and 20 ng ml−1bFGF (c,d). Inserts indshow analysis of expression of indicated markers by flow cytometry; (e) flow cytometric analysis of mesodermal, endothelial and haematopoietic markers in control hESCs and hESCs transduced with indicated TFs on day 5 post transduction; (f,g) ETV2- and ERG-transduced cells acquire endothelial characteristics as shown by positive VE-cadherin immunostaining, AcLDL uptake (f) and formation of endothelial tubes (g). Inserts infshows analysis of AcLDL uptake by flow cytometry. Scale bar,d,f,g, 100 μm. 1 ; Supplementary Table 1 ). We assumed that the ideal hPSC-based system for a gain-of-function screen for haematopoiesis-inductive factors should meet two major requirements: maintain hPSCs in an undifferentiated state, and support expansion of induced haematopoietic cells. We found that these conditions can be met by maintaining hPSCs as a monolayer on matrigel in a basal growth-factor free mTeSR1 medium supplemented with basic fibroblast growth factor (bFGF) and stem cell factor (SCF) and thrombopoietin (TPO) haematopoietic cytokines. In these conditions, the control hESCs or those transduced with enhanced green fluorescent protein (EGFP) remained visibly undifferentiated and retained surface markers and gene expression profile characteristic of hPSCs, while hESCs transduced with lineage factors successfully obtained their differentiation phenotypes ( Fig. 1a–e and Supplementary Fig. 2 ). Figure 1: Gain-of-function screening in hPSCs. ( a ) Schematic diagram of the screening system; ( b – d ) Flow cytometric and immunofluorescent analysis of expression of pluripotency markers in H1 hESCs growing on matrigel for 5 days in standard conditions in mTeSR1 medium ( b ) and basal growth-factor free TeSR1 medium containing 100 ng ml −1 SCF, 50 ng ml −1 TPO and 20 ng ml −1 bFGF ( c , d ). Inserts in d show analysis of expression of indicated markers by flow cytometry; ( e ) flow cytometric analysis of mesodermal, endothelial and haematopoietic markers in control hESCs and hESCs transduced with indicated TFs on day 5 post transduction; ( f , g ) ETV2- and ERG-transduced cells acquire endothelial characteristics as shown by positive VE-cadherin immunostaining, AcLDL uptake ( f ) and formation of endothelial tubes ( g ). Inserts in f shows analysis of AcLDL uptake by flow cytometry. Scale bar, d , f , g , 100 μm. 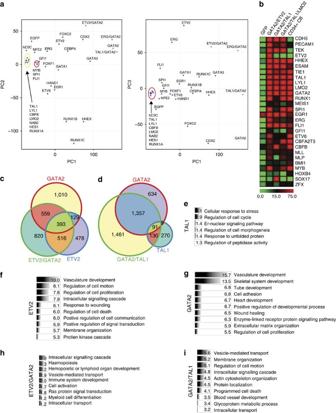Figure 2: Gene expression profiling of hESCs transduced with transcription factors. (a) Principal Component (PC) analysis of global gene expression demonstrates the differences in global gene expression in H1 hESCs transduced with indicated genes. The relative distance is collapsed to two PC1/PC2 and PC1/PC3 dimensions. hESC is non-transduced H1 hESCs control. (b) Heat map shows the expression of genes associated with HSC development, expansion and self-renewal in hESCs transduced with blood-inducing combinations and CD34+cord blood cells. Gene expression is estimated in tpm values. (c,d) The Venn diagrams summarize the number of overlapping and selectively induced genes in hESCs transduced with ETV2, GATA2, TAL1, ETV2/GATA2, and GATA2/TAL1 TFs. Venn diagram shows differentially expressed genes as compared with control hESCs (posterior probability ≥0.99 as determined by EBseq analysis). There is a high overlap between ETV2 and GATA2-induced genes. TAL1 alone has little effect on gene expression; however, in combination with GATA2, TAL1 causes profound changes in the transcriptome. (e–i) The classification of genes induced by indicated combinations of factors into functional categories defined by Gene Ontology (GO) Term using DAVID programme. For GO analysis, each gene set was reduced to include only genes with tpm ≥10 in at least one sample. ETV2/GATA2 and GATA2/TAL1 show genes uniquely induced by two factors together as compared with single factor-transduced cells. The all (TAL1, ETV2/GATA2) or top ten (ETV2, GATA2, GATA2/TAL1) significantly overrepresented categories with FDR below 0.05 (computed according to Benjamini–Hochberg method) are shown. Full size image ETV2 or ERG is sufficient to induce endothelium from hESCs To test the functional capacity of individual genes, we analysed their effect on morphology and expression of following markers by flow cytometry: APLNR and KDR (mesodermal), VE-cadherin, CD34, CD31 and CD73 (endothelial), CD43 and CD45 (haematopoietic) ( Supplementary Table 2 ). Morphological evaluation of the cultures revealed three major effects of TF overexpression: a change in morphology, thereby indicating differentiation; no change in morphology, thus suggesting that cells remain undifferentiated; and early cell death ( Supplementary Table 2 ). Among the 27 tested factors, only 14 triggered morphologic changes in culture without inducing cell death within first 4–5 days after transduction. Although we could not classify the type of formed cells based on morphology alone in most cases, we noticed that ETV2 or ERG-transduced cells acquired the typical morphologic features of endothelial cells ( Supplementary Fig. 2 ). Immunofluorescent and functional analyses revealed that ETV2 and ERG-induced cells expressed VE-cadherin, CD31 and CD34 endothelial markers, uptook AcLDL, and formed vascular tubes in response to vascular endothelial growth factor; which is consistent with the endothelial nature of cells ( Fig. 1e–g ). Gene expression analysis showed that ETV2 or ERG alone are sufficient to induce the expression of almost the entire set of genes required for angiohaematopoietic development, as well as those that are typically expressed in endothelial cells. However, ETV2 and ERG had little effect on the expression of pluripotency genes ( Supplementary Fig. 3a,b ). None of the selected genes were able to induce formation of round blood cells, though we noted weak expression of CD43 by a very few cells following the transduction of cells with ETV2, GATA1 or GATA2 ( Supplementary Table 2 ). Although FOXF1 and HAND1 TFs are shown to be important for lateral plate/extraembryonic mesoderm development in mouse studies [12] , [13] , we found that they did not upregulate the expression of APLNR or KDR pan-mesodermal markers or the genes known to be expressed in lateral plate mesoderm ( Supplementary Fig. 3a ). In contrast, we noticed that GATA2 transduction triggered the expression of TFPA1 , AMOT , APLNR and some other genes associated with endothelial cells, and repressed ESC-specific genes ( Supplementary Fig. 3a,b ). Although GATA1 and GATA3 induced the expression of some endothelial genes similar to GATA2, they also induced the expression of primitive streak genes, and had a less prominent effect on expression of ESC-specific genes, when compared with GATA2 ( Supplementary Fig. 3a ). The Principal Component analysis of the global gene expression and global analysis of changes in gene expression profiles using gene expression dynamics investigator (GEDI) revealed that ETV2, ETV6, ERG, EGR1, CEBPA, FOXC2, HHEX, GATA1, GATA2, GATA3, RUNX1B and RUNX1C caused the most dramatic changes in gene expression, while LMO2 and CBFB TFs, which lack DNA-binding activity, and several DNA-binding molecules including HES1, LYL1, TAL1, MYB, GFI1 and SPI1 had a minimal effect on gene expression in hESCs ( Fig. 2a and Supplementary Fig. 2 ). Figure 2: Gene expression profiling of hESCs transduced with transcription factors. ( a ) Principal Component (PC) analysis of global gene expression demonstrates the differences in global gene expression in H1 hESCs transduced with indicated genes. The relative distance is collapsed to two PC1/PC2 and PC1/PC3 dimensions. hESC is non-transduced H1 hESCs control. ( b ) Heat map shows the expression of genes associated with HSC development, expansion and self-renewal in hESCs transduced with blood-inducing combinations and CD34 + cord blood cells. Gene expression is estimated in tpm values. ( c , d ) The Venn diagrams summarize the number of overlapping and selectively induced genes in hESCs transduced with ETV2, GATA2, TAL1, ETV2/GATA2, and GATA2/TAL1 TFs. Venn diagram shows differentially expressed genes as compared with control hESCs (posterior probability ≥0.99 as determined by EBseq analysis). There is a high overlap between ETV2 and GATA2-induced genes. TAL1 alone has little effect on gene expression; however, in combination with GATA2, TAL1 causes profound changes in the transcriptome. ( e – i ) The classification of genes induced by indicated combinations of factors into functional categories defined by Gene Ontology (GO) Term using DAVID programme. For GO analysis, each gene set was reduced to include only genes with tpm ≥10 in at least one sample. ETV2/GATA2 and GATA2/TAL1 show genes uniquely induced by two factors together as compared with single factor-transduced cells. The all (TAL1, ETV2/GATA2) or top ten (ETV2, GATA2, GATA2/TAL1) significantly overrepresented categories with FDR below 0.05 (computed according to Benjamini–Hochberg method) are shown. Full size image ETV2 and GATA2 induce pan-myeloid hematoendothelial program Accumulated knowledge strongly indicates that blood formation in the embryo proceeds through haemogenic endothelial intermediates [7] , [8] , [9] . Therefore, we decided to test whether the addition of known haematopoietic factors to ETV2 or ERG endothelium-inductive factors would be sufficient to generate endothelium with haemogenic potential. Given the well-established role of GATA2 and GATA1 factors in haematopoietic development, we selected these TFs as a first choice. In fact, transduction of hESCs with ETV2 and GATA2 led to the formation of round CD43 + blood cells with robust CFC potential, while hESCs transduced with ETV2 alone occasionally produced very few small colonies of macrophages and erythroid cells ( Fig. 3a–c ). In clonogenic cultures, ETV2/GATA2-transduced cells formed typical erythroid (CFC-E), macrophage (CFC-M), and large (greater than 0.5 mm in diameter) high proliferative potential colonies (CFC-HPP). Most of the HPP colonies were composed of immature granulocytic and monocytic cells ( Fig. 3b ), but some colonies showed more mature myeloid cells with erythroid and megakaryocytic cells. Cells collected from clonogenic cultures of ETV2/GATA2-transduced hESCs vigorously proliferated in serum-containing medium with haematopoietic cytokines. 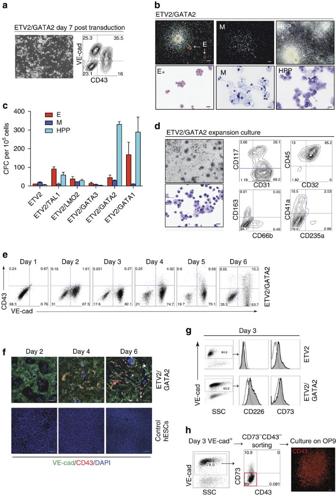Figure 3: Haematopoietic differentiation of hESCs induced by ETV2 and GATA2. (a) Cell morphology and flow cytometric analysis of ETV2/GATA2-transduced H1 hESCs on day 7 post transduction. Scale bar, 100 μm. (b) Types of haematopoietic colonies formed by hESCs on day 7 post transduction with ETV2/GATA2. Erythroid colonies (E); macrophage colonies (M); high proliferative potential myeloid colonies (HPP). Scale bar for CFC assay, 250 μm; cytospins, 20 μm. (c) CFC potential of cells transduced with ETV2 alone and indicated TF combinations. Error bars represent s.e.m. from three to five independent experiments. (d) Phase-contrast photograph of the culture, Wright-stained cytospin and fluorescence-activated cell sorting analysis of ETV2/GATA2-induced haematopoietic cells grown in suspension culture for 14 days in medium supplemented with fetal bovine serum and 100 ng ml−1SCF, 10 ng ml−1IL3, 20 ng ml−1IL6, 10 ng ml−1GM-CSF, 20 ng ml−1G-CSF and 3 u ml−1EPO. (e) Kinetic analysis of VE-cadherin and CD43 expression during direct ETV2/GATA2 programing of H1 hESCs by flow cytometry. (f) VE-cadherin and CD43 immunofluorescent staining of untreated control hESCs and hESCs transduced with ETV2/GATA2 at different time points after transduction. Scale bars, 100 μm. (g) Expression of markers of associated with haemogenic and non-haemogenic endothelium by VE-cadherin+cells emerging on day 3 post transduction with indicated TFs. Histograms show expression of CD226 and CD73 by VE-cadherin-gated cells. Endothelial cells induced by ETV2 alone have CD226−CD73+phenotype associated with non-haemogenic endothelial cells, while ETV2/GATA2 induced endothelium have CD226+CD73−phenotype associated with haemogenic endothelium10. (h) Haematopoietic potential of VE-cadherin+CD43−CD73−endothelial cells isolated from programing cultures. On day 3 after transduction with ETV2/GATA2, VE-cadherin+CD43−CD73−cells were isolated by sorting and cultured on OP9 to assess the haematopoietic potential by counting CD43+haematopoietic colonies using immunofluorescent staining. Blue and red rectangles show position of gates used for cell sorting. Scale bar, 100 μm. After 7 days of expansion, we were able to obtain 24 million CD43 + cells from one million ETV2/GATA2-transduced undifferentiated H1 hESCs ( Supplementary Table 3 ). Flow cytometric analysis of expansion cultures revealed all types of myeloid cells, including CD31 + CD117 + mast cells, CD45 + CD32 + myelomonocytic cells, CD163 + macrophages, CD66b + granulocytes, CD41a + megakaryocytic and CD235a + erythroid cells, thereby indicating that GATA2 and ETV2 induce pan-myeloid haematopoiesis from hESCs ( Fig. 3d ). GATA1 in combination with ETV2 induced a spectrum of haematopoietic colonies similar to GATA2/ETV2 combination, though we noticed an increase in the number of erythroid colonies with ETV2/GATA1 as compared with ETV2/GATA2-transduced cells ( Fig. 3c ). Transduction of cells with ETV2 and GATA3, or TAL1 or LMO2 induced far fewer haematopoietic CFCs and CD43 + cells as compared with ETV2 with GATA2, or GATA1 combinations ( Fig. 3c and Supplementary Fig. 4a ). The addition of other critical haematopoiesis-associated factors, such as TAL1 and LMO2, on top of the ETV2/GATA2 combination, did not substantially change the spectrum of haematopoietic programming ( Supplementary Fig. 4b ). We also found that haematopoiesis can be initiated by transducing cells with ERG together with GATA2 or TAL1 plus LMO2 ( Supplementary Fig. 4b ). However, these combinations induced a very few CFCs most of which were erythroid. Figure 3: Haematopoietic differentiation of hESCs induced by ETV2 and GATA2. ( a ) Cell morphology and flow cytometric analysis of ETV2/GATA2-transduced H1 hESCs on day 7 post transduction. Scale bar, 100 μm. ( b ) Types of haematopoietic colonies formed by hESCs on day 7 post transduction with ETV2/GATA2. Erythroid colonies (E); macrophage colonies (M); high proliferative potential myeloid colonies (HPP). Scale bar for CFC assay, 250 μm; cytospins, 20 μm. ( c ) CFC potential of cells transduced with ETV2 alone and indicated TF combinations. Error bars represent s.e.m. from three to five independent experiments. ( d ) Phase-contrast photograph of the culture, Wright-stained cytospin and fluorescence-activated cell sorting analysis of ETV2/GATA2-induced haematopoietic cells grown in suspension culture for 14 days in medium supplemented with fetal bovine serum and 100 ng ml −1 SCF, 10 ng ml −1 IL3, 20 ng ml −1 IL6, 10 ng ml −1 GM-CSF, 20 ng ml −1 G-CSF and 3 u ml −1 EPO. ( e ) Kinetic analysis of VE-cadherin and CD43 expression during direct ETV2/GATA2 programing of H1 hESCs by flow cytometry. ( f ) VE-cadherin and CD43 immunofluorescent staining of untreated control hESCs and hESCs transduced with ETV2/GATA2 at different time points after transduction. Scale bars, 100 μm. ( g ) Expression of markers of associated with haemogenic and non-haemogenic endothelium by VE-cadherin + cells emerging on day 3 post transduction with indicated TFs. Histograms show expression of CD226 and CD73 by VE-cadherin-gated cells. Endothelial cells induced by ETV2 alone have CD226 − CD73 + phenotype associated with non-haemogenic endothelial cells, while ETV2/GATA2 induced endothelium have CD226 + CD73 − phenotype associated with haemogenic endothelium [10] . ( h ) Haematopoietic potential of VE-cadherin + CD43 − CD73 − endothelial cells isolated from programing cultures. On day 3 after transduction with ETV2/GATA2, VE-cadherin + CD43 − CD73 − cells were isolated by sorting and cultured on OP9 to assess the haematopoietic potential by counting CD43 + haematopoietic colonies using immunofluorescent staining. Blue and red rectangles show position of gates used for cell sorting. Scale bar, 100 μm. Full size image On the basis of these observations, we concluded that ETV2 and GATA2 represent the most optimal combination of TFs for the induction of a robust multilineage haematopoiesis from hESCs, and therefore selected this combination for more detailed analysis. Gene expression profiling revealed that combining ETV2 with GATA2 was sufficient to activate almost the entire spectrum of genes essential for haematopoiesis, including MYB, RUNX1, CBFB and VAV1 genes critical for definitive haematopoiesis, as well as genes associated with myeloid, lymphoid and erythroid lineages ( Fig. 2b ; Supplementary Fig. 5a ). Compared with ETV2 or GATA2 alone, the ETV2/GATA2 combination uniquely induced the expression of 820 genes enriched in the intracellular signalling cascade, haematopoiesis, immune system development, myeloid differentiation and RAS protein signal transduction functional GO categories ( Fig. 2c,h ), consistent with the induction of functional haematopoietic cells by these factors. Kinetic analysis of blood formation by ETV2 and GATA2-transduced cells revealed that haematopoietic development from hESCs proceeds through the endothelial stage. As shown in Supplementary Fig. 5b , the ETV2/GATA2 combination quickly induced CDH5 and PECAM1 endothelial genes in hESCs on day 2 post transduction. The upregulation of CDH5 and PECAM1 was not preceded by substantial and synchronized upregulation of primitive streak and lateral plate mesoderm genes on day 1 post transduction, thus suggesting that ETV2/GATA2 may directly induce the endothelial programme in hESCs bypassing mesodermal stage. The onset of endothelial gene expression was accompanied by induction of the master regulator of definitive haematopoiesis, RUNX1 . Microscopic examination and immunofluorescent staining of cultures revealed that 2–3 days after ETV2 and GATA2 transduction, hESCs acquired VE-cadherin expression and typical morphological features of endothelial cells, similar to ETV2-transduced hESCs ( Fig. 3e,f ). However, in contrast to ETV2 alone, endothelial cells induced after 3 days of ETV2/GATA2 transduction expressed CD226 and lacked CD73 ( Fig. 3g ), that is, displayed phenotypic features that distinguish haemogenic endothelium from non-haemogenic one [10] . The following next 2 days of culture, we observed a transition of endothelial cells into round CD43 + haematopoietic cells, thereby indicating that ETV2 and GATA2 overexpression directly induces formation of endothelial cells with haemogenic properties that subsequently give rise to blood cells ( Fig. 3f and Supplementary Movie 1 ). When VE-cadherin + CD43 − CD73 − cells were collected from ETV2/GATA2-transduced cultures before the detection of CD43 expression (day 3) and cultured on OP9, they generated colonies composed of round CD43 + haematopoietic cells ( Fig. 3h ) at a frequency 501.0±128.4 colonies per 10 5 plated VE-cadherin + CD43 − CD73 − cells. In contrast, VE-cadherin + cells isolated from cultures transduced with ETV2 alone essentially failed to produce CD43 + haematopoietic colonies on OP9 (<2 colonies per 10 5 plated cells). These findings indicate that VE-cadherin + CD43 − CD73 − cells induced by ETV2/GATA2 have functional potentials similar to haemogenic endothelium generated from hESC by differentiation on OP9 (ref. 10 ). GATA2 and TAL1 induce an erythro-megakaryocytic hematoendothelial program Although the basic helix–loop–helix TF TAL1 is a well-known key regulator of haematopoiesis and vasculogenesis [14] , [15] , overexpression of TAL1 alone induced minimal changes in the hESC transcriptome ( Fig. 2a,d ; Supplementary Fig. 2 ) and was not able to induce the formation of endothelium or blood cells from hESCs ( Fig. 1e ). When added to ETV2, TAL1 induced only a few haematopoietic colonies and CD43 + cells ( Fig. 3c and Supplementary Fig. 4a ), while cotransduction of TAL1 with GATA2 efficiently induced the formation of CD43 + haematopoietic progenitors ( Fig. 4a,b ), similar to the ETV2/GATA2 combination. However, in contrast to ETV2/GATA2 combination, haematopoiesis in GATA2/TAL1-transduced cultures was restricted to erythroid and megakaryocytic cells, with the exception of a few macrophages ( Fig. 4b,f ). In tandem with TAL1, GATA2 was essential for the induction of haematopoiesis and could not be replaced with GATA1. When hESCs were transduced with the GATA1/TAL1 combination, they slightly upregulated expression of VE-cadherin and CD43 within the first 4–5 days of culture, but failed to produce a significant number of CFCs afterward ( Fig. 4f ). 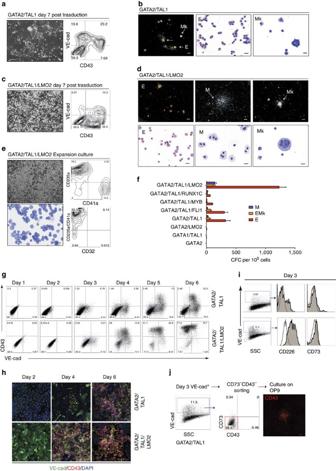Figure 4: Haematopoietic differentiation of hESCs induced by GATA2 and TAL1. (a) Cell morphology and flow cytometric analysis of H1 hESCs differentiated by expression of GATA2 and TAL1 on day 7 post transduction. (b) Types of haematopoietic colonies formed by GATA2 and TAL1 differentiated cells on day 7 post transduction. Erythroid colonies (E); macrophage colonies (M); megakaryocytic colonies (Mk). Scale bar for CFC assay, 250 μm; for cytospins, 20 μm. (c) Cell morphology and flow cytometric analysis of H1 hESCs differentiated by expression of GATA2/TAL1/LMO2 on day 7 post transduction. (d) Types of haematopoietic colonies formed by GATA2/TAL1/LMO2 differentiated cells on day 7 post transduction. Scale bar for CFC assay, 250 μm; for cytospins, 20 μm. (e) Phenotypic characterization of GATA2/TAL1/LMO2-induced haematopoietic cells grown in SFEM serum-free medium supplemented with 100 ng ml−1SCF, 50 ng ml−1TPO, 3 u ml−1EPO and 20 ng ml−1bFGF for 14 days. (f) CFC potential of hESCs transduced with GATA2-based combinations. Error bars represent s.e.m. from three experiments. (g) Kinetic analysis of VE-cadherin and CD43 expression by flow cytometry following transduction of H1 hESCs with indicated combinations of TFs. (h) VE-cadherin and CD43 immunofluorescent staining of hESCs transduced with indicated TFs at different time points after transduction. Scale bars, 100 μm. (i) Expression of markers of associated with haemogenic and non-haemogenic endothelium by VE-cadherin+cells emerging on day 3 post transduction with GATA2/TAL1 (upper panels) and GATA2/TAL1/LMO2 (lower panels). Histograms show expression of CD226 and CD73 by VE-cadherin-gated cells. Endothelial cells induced by GATA2/TAL1 and GATA2/TAL1/LMO2 shows CD226+CD73−phenotype associated with haemogenic endothelium10. (j) Haematopoietic potential of VE-cadherin+CD43−CD73−endothelial cells isolated from GATA2/TAL1 programing cultures. On day 3 after transduction with GATA2/TAL1 or ETV2/GATA2, VE-cadherin+CD43−CD73−cells were isolated by sorting and cultured on OP9 to assess the haematopoietic potential by counting CD43+haematopoietic colonies using immunofluorescent staining. Blue and red rectangles show position of gates used for cell sorting. Scale bar, 100 μm. Figure 4: Haematopoietic differentiation of hESCs induced by GATA2 and TAL1. ( a ) Cell morphology and flow cytometric analysis of H1 hESCs differentiated by expression of GATA2 and TAL1 on day 7 post transduction. ( b ) Types of haematopoietic colonies formed by GATA2 and TAL1 differentiated cells on day 7 post transduction. Erythroid colonies (E); macrophage colonies (M); megakaryocytic colonies (Mk). Scale bar for CFC assay, 250 μm; for cytospins, 20 μm. ( c ) Cell morphology and flow cytometric analysis of H1 hESCs differentiated by expression of GATA2/TAL1/LMO2 on day 7 post transduction. ( d ) Types of haematopoietic colonies formed by GATA2/TAL1/LMO2 differentiated cells on day 7 post transduction. Scale bar for CFC assay, 250 μm; for cytospins, 20 μm. ( e ) Phenotypic characterization of GATA2/TAL1/LMO2-induced haematopoietic cells grown in SFEM serum-free medium supplemented with 100 ng ml −1 SCF, 50 ng ml −1 TPO, 3 u ml −1 EPO and 20 ng ml −1 bFGF for 14 days. ( f ) CFC potential of hESCs transduced with GATA2-based combinations. Error bars represent s.e.m. from three experiments. ( g ) Kinetic analysis of VE-cadherin and CD43 expression by flow cytometry following transduction of H1 hESCs with indicated combinations of TFs. ( h ) VE-cadherin and CD43 immunofluorescent staining of hESCs transduced with indicated TFs at different time points after transduction. Scale bars, 100 μm. ( i ) Expression of markers of associated with haemogenic and non-haemogenic endothelium by VE-cadherin + cells emerging on day 3 post transduction with GATA2/TAL1 (upper panels) and GATA2/TAL1/LMO2 (lower panels). Histograms show expression of CD226 and CD73 by VE-cadherin-gated cells. Endothelial cells induced by GATA2/TAL1 and GATA2/TAL1/LMO2 shows CD226 + CD73 − phenotype associated with haemogenic endothelium [10] . ( j ) Haematopoietic potential of VE-cadherin + CD43 − CD73 − endothelial cells isolated from GATA2/TAL1 programing cultures. On day 3 after transduction with GATA2/TAL1 or ETV2/GATA2, VE-cadherin + CD43 − CD73 − cells were isolated by sorting and cultured on OP9 to assess the haematopoietic potential by counting CD43 + haematopoietic colonies using immunofluorescent staining. Blue and red rectangles show position of gates used for cell sorting. Scale bar, 100 μm. Full size image Since overexpression of TAL1 and GATA2 induced mostly erythroid and megakaryocytic lineages with very few macrophage CFCs, we tested whether the addition of other factors to these combinations would promote multilineage haematopoiesis. As shown in Fig. 4f , the addition of either MYB or RUNX1C factors that are critical for definitive haematopoiesis to GATA2/TAL1 combination was not able to induce the robust myeloid haematopoiesis as was seen with ETV2/GATA2-transduced cells. Likewise, the addition of another ETS TF FLI1 failed to promote myeloid development, indicating that GATA2 and TAL1 combination ‘locked’ cells to erythroid and megakaryocytic lineages. The addition of LMO2 to the GATA2/TAL1 combination dramatically increased haematopoiesis, without significant changes in the spectrum of haematopoietic colonies ( Fig. 4c,d,f ). GATA2/TAL1/LMO2-transduced cells collected from clonogenic cultures robustly expanded in suspension cultures with cytokines. After 7 days of expansion, we were able to obtain 33 million CD43 + cells from one million transduced H1 hESCs. Flow cytometric analysis demonstrated that expansion cultures generated almost exclusively CD235a + erythroid and CD41a + megakaryocytic cells and no CD32 + myelomonocytic cells ( Fig. 4e ), thus confirming the restricted differentiation potential of cells generated from hESCs using these TFs. In cultures transduced with GATA2 and TAL1, the formation of CD43 + round blood cells was preceded by upregulation of VE-cadherin expression ( Fig. 4g,h and Supplementary Movie 2 ), thus indicating that CD43 + cells generated with these two factors, similar to ETV2 and GATA2-transduced cells, arose from endothelial cells through endothelial–haematopoietic transition. Endothelial cells induced by GATA2 and TAL1 on day three of culture, had both the phenotypic and functional features of haemogenic endothelium, that is, they expressed CD226, lacked CD73 ( Fig. 4i ) and were capable of forming of CD43 + blood colonies after culture on OP9 ( Fig. 4j ) at a frequency of 35.6±8.6 colonies per 10 5 plated VE-cadherin + CD43 − CD73 − cells. Transduction of hESCs with the GATA2/TAL1/LMO2 combination, accelerated transition of hESCs into round CD43 + haematopoietic cells with early activation of RUNX1 expression ( Supplementary Fig. 5b ), early appearance of CD43 + VE-cadherin − cells and a markedly contracted endothelial stage of development ( Fig. 4g,h ). Taken together, these observations suggest that GATA2 and TAL1 are critical TFs for specifying hESCs to erythro-megakaryocytic progenitors through haemogenic endothelium intermediates. Induction of hematopoiesis in various hPSCs and by using modified mRNA To determine whether the identified sets of transcriptional regulators were capable of inducing the haematopoietic programme in hPSCs other than H1 hESCs, we overexpressed ETV2/GATA2 or GATA2/TAL1/LMO2 in H9 hESCs and two fibroblast-derived iPSCs. Although yields of blood cells varied between different hPSCs ( Supplementary Table 3 ), the pattern of haematopoietic programming with both combinations of TFs was reliably consistent across all tested cell lines ( Fig. 5a–c ). ETV2 and GATA2 induced pan-myeloid haematopoiesis, including CD32 + myelomonocytic and CD235a + and CD41a + erythroid and megakaryocytic cells, while the TAL1/GATA2/LMO2 combination induced predominantly the erythroid and megakaryocytic cells, but not CD32 + myelomonocytic cells. 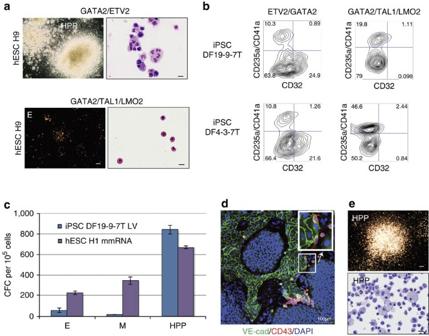Figure 5: Direct haematopoietic programming of various hPSCs using lentiviral vectors and mmRNA. (a) CFCs developed from H9 hESCs 7 days after enforced expression of ETV2/GATA2 and GATA2/TAL1/LMO2. (b) Fluorescence-activated cell sorting analysis of ETV2/GATA2 and GATA2/TAL1/LMO2-transduced iPSC lines DF-19-9-7T and DF-4-3-7T after expansion in suspension cultures in the presence of haematopoietic cytokines (14 day post transduction). (c) CFC potential of DF19-9-7T hiPSCs transduced with ETV2 and GATA2 lentiviral vectors (LV) and H1 hESCs transfected with ETV2 and GATA2 mmRNA. Error bars represent s.e.m. from three experiments. (d) Confocal image of H1 hESC culture 5 days after transduction with ETV2/GATA2 mmRNA. Insert shows the digital zoom of the area outlined by white rectangle where cells are undergoing endothelial–haematopoietic transition. Scale bar, 100 μm. (e) HPP CFCs induced in H1 hESCs by ETV2/GATA2 mmRNA; CFC assay scale bar, 250 μm, cytospins, 20 μm. Figure 5: Direct haematopoietic programming of various hPSCs using lentiviral vectors and mmRNA. ( a ) CFCs developed from H9 hESCs 7 days after enforced expression of ETV2/GATA2 and GATA2/TAL1/LMO2. ( b ) Fluorescence-activated cell sorting analysis of ETV2/GATA2 and GATA2/TAL1/LMO2-transduced iPSC lines DF-19-9-7T and DF-4-3-7T after expansion in suspension cultures in the presence of haematopoietic cytokines (14 day post transduction). ( c ) CFC potential of DF19-9-7T hiPSCs transduced with ETV2 and GATA2 lentiviral vectors (LV) and H1 hESCs transfected with ETV2 and GATA2 mmRNA. Error bars represent s.e.m. from three experiments. ( d ) Confocal image of H1 hESC culture 5 days after transduction with ETV2/GATA2 mmRNA. Insert shows the digital zoom of the area outlined by white rectangle where cells are undergoing endothelial–haematopoietic transition. Scale bar, 100 μm. ( e ) HPP CFCs induced in H1 hESCs by ETV2/GATA2 mmRNA; CFC assay scale bar, 250 μm, cytospins, 20 μm. Full size image To find out whether the induction of blood formation from hPSCs in our system requires continuous or transient expression of transcriptional regulators, we performed direct programming studies using ETV2 and GATA2-modified mRNA (mmRNA). As shown in Fig. 5c–e , transfection of H1 hESCs with ETV2 and GATA2 mmRNA induced the haematoendothelial programme and robust formation of the same spectrum of CFCs as we observed with lentivirus-transduced cells. Using mmRNA transfection, we were able to generate 11.6 million CD43 + cells from one million H1 hESCs following transfection and 7-day expansion. These studies provide the evidence that brief expression of ETV2 and GATA2 is indeed sufficient to commit the hPSCs to blood fate. Using a gain-of-function genetic screen, we identified ETV2 and GATA2 as the most critical TFs required for the induction of the haemogenic endothelium with pan-myeloid potential from hESCs. ETV2 belongs to the ETS family of TFs, which also includes ERG, and plays a critical role in endothelial development [16] . Gain-of-function experiments in Xenopus and zebrafish embryos have demonstrated that ETV2 and ERG are capable of inducing ectopic endothelial differentiation [17] , [18] , [19] . ETV2 and ERG are also essential for establishing definitive haematopoiesis and the proper function of adult HSCs [20] , [21] , [22] , [23] . We found that ectopic expression of ETV2 and ERG in undifferentiated hESCs upregulates the expression of genes associated with angiohaematopoietic development and typical endothelial genes resulting in the formation of endothelial cells. Although overexpression of ETV2 or ERG alone induced the expression of endogenous FLI1, GATA2 and TAL1 genes that form the kernel of the gene regulatory network in developing HSCs [24] , ETV2 or ERG-induced endothelium was lacking significant blood-forming activity. Overexpressing GATA2 in addition to ETV2 was essential to induce endothelial cells with robust blood-forming potential. The ERG-mediated endothelial programme was much less susceptible to haemoinductive effect of GATA2, indicating a unique requirement for synergistic action of ETV2 and GATA2 TFs for optimal activation of pan-myeloid haematopoietic programme from hPSCs. Although prior studies in mouse ESCs have shown the synergistic role of Etv2 and Gata2 in haematoendothelial specification from mesoderm [25] , [26] , we have revealed for the first time that these two factors are sufficient to directly induce haematoendothelial programme from undifferentiated PSCs in humans. Mouse studies have demonstrated that Tal1 controls the expression of several important haematopoietic regulators, including Runx1, Erg, Gfi1b and Gata2 among others [27] . Tal1 is considered as a key component of the regulatory network controlling HSC specification [24] . Tal1 also plays an important role in vascular development and is required for embryonic vascular remodelling [15] , [28] and haemangioblast specification [29] , [30] . Enforced expression of Tal1 in normal zebrafish embryos causes overproduction of endothelial and haematopoietic cells [30] . However, enforced TAL1 expression in hESCs induced only minimal changes in the transcriptome and failed to trigger morphologic changes, thereby suggesting that TAL1 alone can’t create a TF network to direct the activation of the angiogenic programme in hESCs as we observed with ETV2 and ERG. Yet, TAL1 was capable of triggering blood development when coexpressed together with ETV2 or GATA2. ETV2/TAL1 combination induced pan-myeloid haematopoiesis in hESC cultures similar to cultures transduced with ETV2 and GATA2, but with much less efficiency. Enforced expression of TAL1 with GATA2 induced robust haematopoiesis, but it produced mostly erythroid and megakaryocytic cells. Interestingly, haematopoietic development in GATA2/TAL1-transduced cultures proceeded through the haemogenic endothelium stage similar to cultures transduced with ETV2 and GATA2, which generated pan-myeloid CFCs. These observations suggest that two groups transcriptional regulators can trigger activation of TF network leading to formation of haemogenic endothelium with different functional capacities: GATA2/TAL1-induced haemogenic endothelium with restricted erythro-megakaryocytic and macrophage potential, and ETV2/GATA2-induced endothelium with pan-myeloid potential. Although the concept of haemogenic endothelium was developed by observing HSC and blood formation from the aortic endothelium in the aorta-gonad-mesonephros region, it has become clear that endothelium in other embryonic and extraembryonic sites possess haemogenic potential. Among these sites are the vitelline and umbilical arteries [31] , placenta [32] , head vasculature [33] , endocardium [34] and nascent yolk sac capillaries [35] . However, not all haemogenic endothelium has the capacity to produce HSCs. In the aorta-gonad-mesonephros region, HSCs are restricted to the ventral wall of the dorsal aorta, while haematopoietic progenitors without HSC potential can be found at several other sites within the embryonic aorta [31] , [36] , underscoring that haemogenic potential of the aortic endothelium is variable. Recently, Chen et al . [37] identified at least two distinct types of haemogenic endothelium in the embryo, implying that specification of the haematopoietic programme may take place at the haemogenic endothelium stage. Further support for this concept came from clonal functional and molecular analyses of haemogenic endothelium undergoing endothelial–haematopoietic transition in mouse embryo which found that the haematopoietic programme is already initiated in cells embedded in the endothelial layer. [38] Our present studies have demonstrated that haemogenic endothelium with distinct haematopoietic programs can be induced from hPSCs, and that different groups of TFs are required for the induction of haemogenic endothelium with pan-myeloid or restricted erythro-megakaryocytic programme. These observations strongly support the concept of heterogeneity of haemogenic endothelium and provide additional evidence that lineage-specific haematopoietic programs from hPSCs can be established at the haemogenic endothelium stage. Production of haematopoietic cells with long-term repopulating potential from hPSCs remains a significant challenge. Although we demonstrated that ETV2/GATA2 combination induces robust formation of multipotential CFCs, we failed to detect meaningful engraftment of these cells in NOD/SCID/IL2Rγ −/− mice, suggesting that TF-induced cells have similar properties to haematopoietic progenitors obtained from hPSCs using conventional differentiation methods. Nevertheless, identification of critical pathways leading to the formation of distinct types of haemogenic endothelium in the current study provided a novel experimental platform to further explore the transcriptional programme in hPSCs required for activation of the self-renewal programme in hPSC-derived haematopoietic cells. Recently, studies by Pereira et al . [39] have shown that the haemogenic programme can be induced in mouse fibroblasts via the overexpression of Gata2, Gfi1b, cFos, and Etv6, thus indicating the feasibility of generating a haematopoietic hierarchy by bypassing the pluripotency stage. Pursuing both approaches to generating blood cells, pluripotent stem cell-based and direct reprogramming of somatic cells, will be essential to better understand the genetic and epigenetic factors governing haematopoietic fate determination and the self-renewal programme, and will contribute substantially to the ultimate goal of developing technologies for in vivo production of HSCs for clinical purposes. Cloning of selected genes and virus production Open reading frames of selected genes were amplified from cDNA of H1 hESCs differentiated in coculture with OP9, or from full-length cDNAs clones obtained from Open BioSystems (Pittsburgh, PA) and Gene Copoeia Inc. (Rockville, MD). After sequence verification, open reading frames were subcloned into pSIN/EF1α-IRES-Puro lentiviral expression vector. Virus production was carried out by calcium phosphate transfection of Lenti-X 293T cells (Clontech, Mountain View, CA). Packaged lentiviral units were concentrated either on ethylene oxide-sterilized Centricon Plus-70 or Amicon Ultra-15 Centrifugal Filter Units (Millipore, Billerica, MA), or by ultracentrifugation at 33,000 r.p.m. for 2.5 h (Beckman Optima XL-A analytical ultracentrifuge, Beckman Coulter, Inc., USA) and resuspended in 1% bovine serum albumin in phosphate-buffered saline (PBS). Amount of Infectious Units per ml of viral concentrate was assessed by transduction and puromycin selection of HeLa cells with a working puromycin concentration of 1 μg ml −1 . Successful transduction was confirmed by demonstration of virus integration by genomic PCR and transgene mRNA expression by RNAseq analysis. Cell culture and hPSCs transductions Irradiated mouse embryonic fibroblasts, human embryonic stem cell lines H1 (WA01) and H9 (WA09), fibroblast-derived human-induced pluripotent stem cell lines DF-19-9-7T and DF-4-3-7T were obtained from WiCell (Madison, WI). hESCs and hiPSCs were maintained on mouse embryonic fibroblasts in DMEM/F12 basal medium supplemented with 20% of KnockOut Serum Replacement, 0.1 mM non-essential amino acids, 0.1 mM β-mercaptoethanol, 1 mM L-Glutamine (Gibco, Invitrogen, Carlsbad, CA) and 4 ng ml −1 of bFGF. Before lentiviral transduction experiments, pluripotent stem cells were grown on Matrigel (BD Biosciences, Bedford, MA) in feeder-free conditions in chemically defined mTeSR 1 medium (StemCell Technologies, Vancouver, Canada) from two to five passages. hPSCs monolayers at 70% of confluence were washed with PBS and dissociated to a single cell suspension by incubation with StemPro Accutase (Invitrogen, Carlsbad, CA). At all intermediate steps of hPSCs collection, cells were kept on ice in mTeSR1 medium containing 10 μg ml −1 of Y-27632 ROCK Inhibitor (Stemgent, Cambridge, MA). 0.7-1 × 10 6 of dissociated cells were mixed with concentrated viral medium (multiplicity of infection=1–5) in 1 ml of mTeSR1 containing 10 μg ml −1 Y-27632 ROCK Inhibitor and 6 μg ml −1 of polybrene (Sigma). hPSCs suspensions containing virus were plated on six-well matrigel-coated plates, and incubated for 12 h in standard conditions (37 °C, 5% CO 2 , >95% humidity). After 12 h, virus-containing medium was replaced with fresh mTeSR1 medium. On day 1 after transduction, regular mTeSR1 was replaced with basal mTeSR1 medium supplemented with cytokines SCF (100 ng ml −1 ), TPO (50 ng ml −1 ) and bFGF (20 ng ml −1 ; PeproTech, Rocky Hill, NJ). Since the presence of puromycin in differentiation cultures had a little effect on the outcomes of cellular transductions, hPSCs differentiation experiments were performed without antibiotic selection. Cells transduced with a single factor were maintained in indicated conditions from 3 to 7 days, depending on their survival and growth, and collected for analysis ( Supplementary Table 2 ). Cell transduced with different combinations of factors were collected after seven days of culture. Nucleofection with modified mRNAs ETV2 and GATA2-modified messenger RNAs (mmRNAs) were kindly provided by NHLBI Progenitor Biology Consortium RNA Core ( http://www.progenitorcells.org/content/requesting-rnacore-service ). Nucleofection of H1 hESCs with modified messenger RNAs (mmRNAs) was performed using Amaxa Human Stem Cell Nucleofector Kit 2 (Lonza). Before nucleofection, cells were washed with PBS and dissociated to a single cell suspension using StemPro Accutase (Invitrogen) as described above. For one nucleofection reaction, 2 × 10 6 cells were resuspended in 100 μl of nucleofection reagent containing mmRNA (1.75 μg of both GATA2 and ETV2; 3.5 μg in total), transferred immediately to nucleofection cuvette and transfected using B-016 programme on the Amaxa Nucleofector II (Lonza). After the procedure, cells were resuspended in 500 μl of mTeSR1 medium with Y-27632 ROCK inhibitor and transfered to matrigel coated six-well plates containing 2 ml of mTeSR1 medium. After a 24-h incubation, cells were collected and transfected a second time as described above. Twenty-four hours after the second transfection, the medium was change to growth-factor-free basal TeSR1 medium containing SCF (100 ng ml −1 ), TPO (50 ng ml −1 ) and bFGF (20 ng ml −1 ). Immunostaining procedures Expression of cell surface proteins was assessed by routine flow cytometry protocol (FACSCalibur, BD Biosciences). For intracellular staining by FACS, cells were fixed for 10 min at 37 °C in BD Cytofix buffer (BD Biosciences), followed by permeabilzation for 30 min on ice in Perm Buffer III (BD Biosciences). After washing, cells were stained at 4 °C for 2 h with fluorescence-conjugated antibodies. For in situ staining, cell cultures were fixed with 4% paraformaldehyde, permeabilized with 0.05% of Triton X-100 and incubated overnight at 4 °C with primary antibodies, followed by staining with the secondary fluorochrome-labelled antibodies. Intranuclear staining of pluripotency markers was performed by permeabilization with ice-cold 0.2% Triton X-100 in PBS. All antibodies used in this study are listed in Supplementary Table 4 . Images acquired with an inverted Olympus IX71 microscope or Nikon Eclipse Ti-E configured with an A1R confocal system. Haematopoietic colony-forming assay Haematopoietic clonogenic assays were performed using cells collected at day 7 after lentiviral transduction and serum-containing methylcellulose media (MethoCult) supplemented with SCF, G-CSF, GM-CSF, IL3, IL6 and EPO (StemCell Technologies) according to the manufacture’s protocol. Wright staining (Sigma-Aldrich) was used to evaluate the morphology of cells within colonies on cytospins. Endothelial assays To assess endothelial potential, cells were collected on day 7 post transduction and placed on fibronectin-coated six-well plates (hFibronectin, BD) supplemented with complete Endothelial Cell Medium ECM (ScienCell, Carlsbad, CA). Once cells achieve monolayer, they were evaluated for VE-cadherin expression by immunofluorescence, AcLDL uptake and tube formation. For AcLDL uptake assay, cells growing in a monolayer were incubated with 10 μm ml −1 of Alexa-594- or Alexa-488-conjugated AcLDL (Invitrogen) for 4 h at 37 °C followed by fluorescent microscopy or flow cytometric analysis. For vascular tube formation, 2 × 10 4 cells were resuspended in ECM medium (ScienCell) supplemented with 40 ng ml −1 vascular endothelial growth factor (PeproTech) and placed on matrigel matrix. Cells were incubated at 37 °C, 5% CO2 for 18–24 h when tube formation was observed. Evaluation of haemogenic potential of induced endothelium Cells transduced with TFs were collected at day 3 post transduction and labelled with VE-cadherin, CD43 and CD73 antibodies. VE-cadherin + CD43 − CD73 − cells were sorted using FACSAria cell sorter and cultured in a six-well plate (3 × 10 4 cell per well) on OP9 monolayer in αMEM basal medium supplemented with 10% FBS (HyClone), 100 mM monothioglycerol and 50 μg ml −1 of ascorbic acid. After 2 weeks of culture, the formation of blood colonies in cultures was assessed using CD43 immunoflurorescent staining. RNAseq and bioinformatics analysis Cells transduced with single TF were collected on day 3–7 post transduction as indicated in Supplementary Table S2 . Cells transduced with different TF combinations were collected on day 7 after transduction. Cord blood CD34 + cells were obtained from Cincinnati Children's Hospital Medical Center (CCHMC). Total RNA was isolated using RNeasy Micro Kit (Qiagen). Treatment with DNaseI was performed on the column according to the manufacture’s protocol. Purity and integrity of RNA was estimated by the capillary electrophoresis on the Bioanalyzer 2100 (Agilent Technologies, Santa Clara, CA). Samples were then prepared for sequencing using the Illumina TruSeq RNA Sample Preparation Kit v2 (RS-122-2001), according to the manufacturer’s protocol. Final sample libraries were quantitated with the Life Technologies Qubit fluorometer and sequenced on the Illumina HiSeq 2500 (SY-401-1003-PRE). Base-calling and demultiplexing were done with the Illumina Genome Analyzer Casava Software, version 1.8.2. After quality assessment and filtering for adapter molecules and other sequencing artifacts, the remaining sequencing reads were aligned to 19084 RefSeq genes extracted from the Illumina iGenomes annotation, selecting only ‘NM_’ designated genes. Bowtie v 0.12.9 was used, allowing two mismatches in a 28 bp seed, and excluding reads with more than 200 alignments [40] . RSEM v 1.2.3 was used to estimate isoform or gene relative expression levels in units of ‘transcripts per million’ (tpm), as well as ‘expected counts’ (the non-normalized absolute number of reads assigned by RSEM to each isoform per gene). [41] , [42] To determine differentially expressed genes between selected treated samples and H1 hESC controls, the expected counts data were analysed using EBSeq. Genes with a posterior probability ≥0.99 were considered differentially expressed. Venn diagrams were constructed showing the overlap of gene sets identified in each of the treatment samples as ‘Up-regulated’ with respect to the H1 controls. For GO analysis, each gene set was further reduced to include only genes with tpm≥10 in at least one sample. Enrichment of functional categories in the list of responsive genes was computed using the DAVID webservice ( http://david.abcc.ncifcrf.gov/ ) [43] . To visualize the significance of the overrepresentation, negative log 10 of FDRs were plotted as bars, where FDR is computed by DAVID according to the Benjamini–Hotchberg method [44] . To visualize the gene expression levels, a heat map was composed using MultiExperiment Viewer v4.2 ( http://www.tm4.org ). The visualization of global transcriptional signature of cells after transduction with single factor was performed using the Gene Expression Dynamics Inspector (GEDI) plots [45] . Time-lapse microscopy To capture the endothelial–haematopoietic transition, the time-lapse movies were recorded using Nikon Eclipse Ti-E configured with an A1R confocal system and motorized stage (Nikon Instruments Inc., Melville, NY). Cell cultures were washed thoroughly to remove debris, and VE-cadherin-FITC and CD43-PE antibodies were added to a final concentration of 100 ng ml −1 . Presented movies were made on day 3.5 post transduction for GATA2/TAL1-induced cells and on day 4 for GATA2/ETV2-induced cells. Images were acquired using Nikon Elements (NIS-element C) imaging software for every 5 min with CFI Plan Fluor DLL × 20 NA 05 WD 2.1 MM objective (Nikon Instruments Inc.). To convert time-lapse serial images to movies, the Quick-time movies and ImageJ (NIMH, Bethesda, MD) software were applied. How to cite this article: Elcheva, I. et al . Direct induction of haematoendothelial programs in human pluripotent stem cells by transcriptional regulators. Nat. Commun. 5:4372 doi: 10.1038/ncomms5372 (2014). Accession codes : The RNAseq data has been deposited in Gene Expression Omnibus under accession number GSE57395 .